Reactivity mapping with electrochemical gradients for monitoring reactivity at surfaces in space and time Studying and controlling reactions at surfaces is of great fundamental and applied interest in, among others, biology, electronics and catalysis. Because reaction kinetics is different at surfaces compared with solution, frequently, solution-characterization techniques cannot be used. Here we report solution gradients, prepared by electrochemical means, for controlling and monitoring reactivity at surfaces in space and time. As a proof of principle, electrochemically derived gradients of a reaction parameter (pH) and of a catalyst (Cu(I)) have been employed to make surface gradients on the micron scale and to study the kinetics of the (surface-confined) imine hydrolysis and the copper(I)-catalysed azide-alkyne 1,3-dipolar cycloaddition, respectively. For both systems, the kinetic data were spatially visualized in a two-dimensional reactivity map. In the case of the copper(I)-catalysed azide-alkyne 1,3-dipolar cycloaddition, the reaction order (2) was deduced from it. Chemical reactions at surfaces are of great fundamental and applied interest, for example in biology [1] , [2] , electronics [3] and catalysis [4] , [5] , [6] . Investigating and monitoring reactivity is therefore of paramount importance [7] , [8] , [9] to evaluate a surface reaction’s scope and applicability. Monolayers are an excellent platform to investigate interfacial reactions and reactivity because of the ability to precisely control surface composition [7] , [10] , [11] , [12] , [13] . Because reaction kinetics is different at surfaces compared with solution, frequently, solution-characterization techniques cannot be used. Gradients of physicochemical properties, that is, their continuous variation in space and/or time, are of great value both in solution and on surfaces for many applications and systems, such as for the screening of catalysts [14] , [15] and biomaterials [16] , and for studying dynamic phenomena such as the chemotaxis of cells [17] and the motion of water droplets [12] or molecules [18] . Many methods have been developed to create static surface gradient patterns on the sub-mm lengthscale [19] . For the sub-μm lengthscale, not many methods are available to produce such gradients, which would be worthwhile from the perspective of, for example, studying the motion of individual (bio)molecules and the investigation and screening of nanomaterials. None of the existing (sub)μm gradient methods is compatible with switching on/off or dynamically changing gradient properties in time, which has been done at the sub-mm lengthscale for biological surfaces [20] to study cell chemotaxis [21] . This report presents solution gradients, prepared by electrochemical means, for controlling and monitoring reactivity at surfaces in space and time in a high-throughput manner. Because the solution gradient provides a tunable and intrinsically predictable, spatial concentration variation of a chemically reactive species, and therefore of the reaction parameter, the reactions yield micron-scale surface gradients, and the kinetic data are directly correlated with a kinetic model of the surface reaction at hand. In this way, not only kinetic rate constants are obtained but also their spatial variation is directly visualized, yielding a reactivity map, and translated into the reaction rate order. 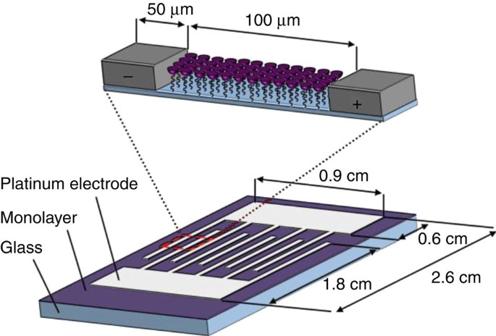Figure 1: Setup of the system. Schematic overview of the setup, showing the dimensions and overall design of the interdigitated electrode array, with which the electrochemically derived gradients are formed. The system Figure 1 shows a schematic overview of the setup, showing the dimensions and overall design. As a proof of principle, electrochemically derived gradients of a reaction parameter ((pH) or concentration of a homogeneous catalyst, Cu(I)) were employed to make surface gradients on the micron scale and to study the kinetics of the (surface-confined) imine hydrolysis and the copper(I)-catalysed azide-alkyne 1,3-dipolar cycloaddition (CuAAC; ‘click’ reaction), respectively. The acid-catalysed imine hydrolysis [22] , [23] belongs to the area of dynamic covalent chemistry [24] , combining the reversible and dynamic properties characteristic of supramolecular chemistry with the strength and robustness of covalent bond chemistry. After introduction of the imine bond in surface chemistry [25] , the imine formation and hydrolysis reactions, owing to their mild reaction conditions, are being used for bioapplications [26] . The second (CuAAC) reaction is a widely used reaction because of its high yield, orthogonality and chemoselectivity [27] , which makes it a useful reaction for surface functionalization [28] . Figure 1: Setup of the system. Schematic overview of the setup, showing the dimensions and overall design of the interdigitated electrode array, with which the electrochemically derived gradients are formed. 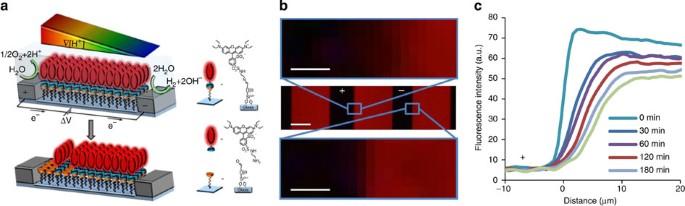Figure 2: Micron-scale surface imine gradient formation by a solution pH gradient. (a) Schematic representation of the electrochemical generation, via the electrolysis of water between interdigitated electrodes, of a solution pH gradient, which is transferred to a surface gradient by means of acid-catalysed imine hydrolysis resulting in a gradient of a surface-bound rhodamine dye. (b) Fluorescence microscopy images showing an overview (centre) and zoom-ins of (top) the generated, surface-bound, imine gradient at the anode (low pH) and of (bottom) an unchanged boundary at the cathode (high pH) after applying the pH gradient for 240 min, 1.6 V, 1 mM, pH 7.1, phosphate buffer and 100 mM Na2SO4(50 μm electrodes, 100 μm gap). Scale bar, 50 μm; 3 μm (zoom-in). (c) Fluorescence intensity profiles visualizing the rhodamine dye gradients directly after hydrolysis close to the anode at different reaction times (raw data). Full size image Imine hydrolysis Figure 2a shows the schematic representation of the imine hydrolysis in an electrochemically produced pH gradient in solution. An amine-functionalized rhodamine dye is immobilized by imine bond formation onto an aldehyde monolayer [29] at a glass surface in between the electrodes of an interdigitated microelectrode array. On top of the full monolayer of the rhodamine dye, a pH gradient is applied [30] , [31] . The pH gradient is generated via the electrolysis of water, thus generating H + and OH − at the anode and cathode, respectively. A phosphate buffer was used to stabilize the pH gradient [30] . Figure 2: Micron-scale surface imine gradient formation by a solution pH gradient. ( a ) Schematic representation of the electrochemical generation, via the electrolysis of water between interdigitated electrodes, of a solution pH gradient, which is transferred to a surface gradient by means of acid-catalysed imine hydrolysis resulting in a gradient of a surface-bound rhodamine dye. ( b ) Fluorescence microscopy images showing an overview (centre) and zoom-ins of (top) the generated, surface-bound, imine gradient at the anode (low pH) and of (bottom) an unchanged boundary at the cathode (high pH) after applying the pH gradient for 240 min, 1.6 V, 1 mM, pH 7.1, phosphate buffer and 100 mM Na 2 SO 4 (50 μm electrodes, 100 μm gap). Scale bar, 50 μm; 3 μm (zoom-in). ( c ) Fluorescence intensity profiles visualizing the rhodamine dye gradients directly after hydrolysis close to the anode at different reaction times (raw data). Full size image A finite-element model was set up to estimate the pH gradient [32] . The modelled pH gradient, as a function of time, is shown in Supplementary Fig. S1 and indicates a pH gradient spanning roughly 1 pH unit. This pH range was confirmed experimentally by monitoring the fluorescence intensity of a pH-dependent dye attached at the glass surface in between the electrodes upon subjecting it to the pH gradient, as shown in Supplementary Figs S2 and S3 . Imine hydrolysis is acid-catalysed and therefore the rhodamine dye is expected to be removed close to the anode while the rate of this reaction is dependent on the pH and thus, in our pH gradient setup, on the distance to the anode. Figure 2b shows a fluorescence microscopy image with an overview of a sample, and zoom-ins of the generated, surface-bound, dye gradient at the anode (low pH) and an unchanged boundary at the cathode (high pH) after applying the pH gradient for 240 min. Figure 2c shows untreated fluorescence intensity profiles near the anode at different reaction times, clearly visualizing the decrease of fluorescence intensity in time close to the anode (low pH), indicating the hydrolysis of the imine bond. Furthermore, Supplementary Fig. S4 shows a zoom-in near the cathode at different reaction times, which shows, as expected, negligible hydrolysis at high pH. The images and profiles show that this system can be used to make surface gradients at the low-micron scale. To prove that hydrolysis is taking place, back to the original aldehyde, the hydrolysed, aldehyde-containing area close to the anode was backfilled by amine-functionalized fluorescein as shown online in Supplementary Fig. S5 . Potentially, silane–silanol bond hydrolysis can be promoted under acidic and alkaline pH. From the estimation of the pH gradient (see above), this effect is negligible at the basic pH side, consistent with Supplementary Fig. S4 . Moreover, physisorption of amine-functionalized fluorescein was found to be negligible as well ( Supplementary Fig. S6 ), which indicates that the observed backfilling can be attributed to the specific binding to reformed aldehyde groups near the anode. The successful imine formation of the fluorescein-labelled amine reagent confirms the reversibility of the platform, and at the same time excludes the darkening occurring near the anode upon hydrolysis to be the result of destruction of the dye or of the reactive monolayer. The results also show that we can reliably make μm-sized surface gradients, with control over on/off and dynamically changing the gradient properties in time, which is not shown before for μm-gradient methods [19] and is worthwhile from the perspective of, for example, studying the motion of individual (bio)molecules and the investigations and screening of nanomaterials. The fluorescence data of the imine hydrolysis, shown in Fig. 2c versus distance, was plotted versus time as shown in Fig. 3a , as a function of the distance from the anode. 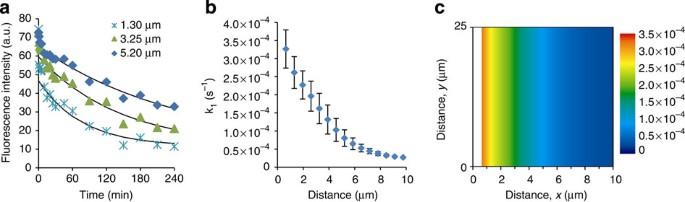Figure 3: Reactivity mapping of the imine hydrolysis reaction. (a) Data and exponential fits (I(t)=(Imax−Io)*e-k1t+Io) of the surface-confined imine hydrolysis at some characteristic distances from the anode (low pH). (b) Resulting (averaged;±1 s.d.) values of the first-order rate constant,k1, of the imine hydrolysis versus distance from the anode. (c) A two-dimensional reactivity map of the imine hydrolysis kinetics showing the (averaged)k1values mapped in space next to an anode (running vertically and ending atx=0). Figure 3a shows representative graphs of the fitted data at three specific distances. These time traces were fitted to an exponential decay function: Figure 3: Reactivity mapping of the imine hydrolysis reaction. ( a ) Data and exponential fits ( I(t) =( I max −I o ) * e - k 1 t + I o ) of the surface-confined imine hydrolysis at some characteristic distances from the anode (low pH). ( b ) Resulting (averaged;±1 s.d.) values of the first-order rate constant, k 1 , of the imine hydrolysis versus distance from the anode. ( c ) A two-dimensional reactivity map of the imine hydrolysis kinetics showing the (averaged) k 1 values mapped in space next to an anode (running vertically and ending at x =0). Full size image where I is the fluorescence intensity (a.u.) at time t (s), I max is the starting fluorescence (a.u. ), I 0 is the background fluorescence (a.u.) and k 1 is the reaction rate constant (s −1 ). Because (i) the reaction mechanism can be assumed to be first-order in imine concentration, (ii) the reverse reaction can be assumed to be absent because of rapid diffusion and dilution of the desorbed rhodamine amine and (iii) the fluorescence intensity can be assumed to be linearly correlated with the imine surface density; k 1 is assumed to be the first-order rate constant of the hydrolysis reaction. The data in Fig. 3a appears to show two-phase kinetics. A two-phase kinetics has been observed before [33] for imine hydrolysis but then a lower initial rate was followed by a faster consecutive reaction. This was attributed to the initially closely packed SAM, which may protect the imine bond from the solution. In our case, however, we may attribute the initially faster hydrolysis to a steeper pH gradient in the beginning as is evident from a higher current (see also Supplementary Fig. S7 ). However, because the pH gradient is not stable in those first few minutes, as is evident from Supplementary Fig. S1 , only the data from 20 min onwards were fitted. For the overall analysis, this is not expected to pose any problem because of the relative timescales between the total hydrolysis period (3 h) versus the start-up phase (10 min). The resulting averaged first-order rate constants for the imine bond hydrolysis versus distance from the anode are shown in Fig. 3b . As expected, k 1 is highest close to the anode, and decreases to a background value that is roughly 15 times lower than close to the anode. Reasons why k 1 does not go to zero can be: (i) the data are uncorrected for bleaching and (ii) the hydrolysis of an imine bond is primarily acid-catalysed but can occur over a large pH range [34] , [35] . Figure 3c shows a reactivity map of the surface-confined imine hydrolysis, with the spatial parameters retained, showing (averaged) k 1 versus distance from the anode ( x axis) and along the anode ( y axis). It is envisaged that also in case of more complex (for example, two-dimensional) gradients, such a graphical representation of kinetic data is powerful and can show interesting kinetic regimes as a function of one or more spatially mapped reaction parameters. Click reaction A schematic representation of the second (CuAAC) reaction studied is shown in Fig. 4a , in which a [Cu(I)] gradient is applied on top of an azide-terminated silane layer that is attached to the glass substrate areas between the electrodes of an interdigitated electrode array. The Cu(I) catalyst is formed in situ by an one-electron reduction of already present Cu(II) [36] , at the cathode (source), whereas oxidation of the generated Cu(I) back to Cu(II) at the anode (sink) makes sure a stable gradient is formed. The solution gradient of [Cu(I)] is then exploited in the electrochemically activated CuAAC (‘e-click’) of an alkyne from solution to the azide monolayer resulting in a surface gradient. The reaction is monitored ex situ via immobilization of an alkyne-modified fluorescein onto the azide-terminated monolayer. The rate of this reaction is expected to be the highest close to the cathode, at which electrode the reduction of Cu(II) to Cu(I) is expected to occur. 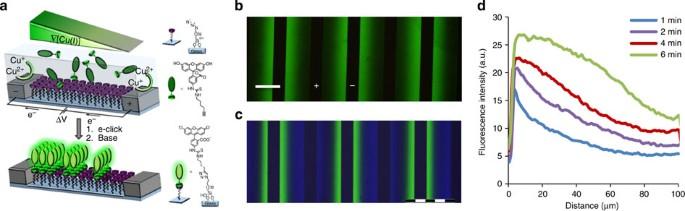Figure 4: Micron-scale surface ‘clicked’ gradient formation via a [Cu(I)] solution gradient. (a) Schematic representation of the electrochemical generation of a [Cu(I)] gradient in solution between the electrodes of an interdigitated electrode array, obtained via the reduction of Cu(II) to Cu(I) and oxidation of the resulting Cu(I) to Cu(II) at the cathode and anode, respectively. This solution gradient is transferred to a surface gradient by means of the electrochemically activated click reaction of a fluorescein-labelled alkyne to an azide monolayer, resulting in a surface-bound fluorescein dye gradient. (b) Fluorescence microscopy image of the resulting surface gradient, 1.0 mM fluorescein alkyne, 1.0 mM CuSO4salt in dimethylsulphoxide,ΔV=1 V, 4 min reaction time (50 μm electrodes, 100 μm gap). Scale bar, 100 μm. (c) Fluorescence microscopy image, after overlay of images made using the green (λexc=495 nm,λem≥520 nm) and blue (λexc=350 nm,λem≥420 nm) filters, of a bi-component surface chemical gradient by means of the ‘e-click’ (2 min) of a fluorescein-labelled alkyne followed by a switch of the polarity of the electrodes and performing a further ‘e-click’ (2 min) of a coumarin-labelled alkyne. Scale bar, 200 μm. (d) Fluorescence intensity profiles versus distance from the cathode visualizing the resulting dye gradient for different reaction times (raw data, obtainedex situ). Figure 4: Micron-scale surface ‘clicked’ gradient formation via a [Cu(I)] solution gradient. ( a ) Schematic representation of the electrochemical generation of a [Cu(I)] gradient in solution between the electrodes of an interdigitated electrode array, obtained via the reduction of Cu(II) to Cu(I) and oxidation of the resulting Cu(I) to Cu(II) at the cathode and anode, respectively. This solution gradient is transferred to a surface gradient by means of the electrochemically activated click reaction of a fluorescein-labelled alkyne to an azide monolayer, resulting in a surface-bound fluorescein dye gradient. ( b ) Fluorescence microscopy image of the resulting surface gradient, 1.0 mM fluorescein alkyne, 1.0 mM CuSO 4 salt in dimethylsulphoxide, ΔV =1 V, 4 min reaction time (50 μm electrodes, 100 μm gap). Scale bar, 100 μm. ( c ) Fluorescence microscopy image, after overlay of images made using the green ( λ exc =495 nm, λ em ≥520 nm) and blue ( λ exc =350 nm, λ em ≥420 nm) filters, of a bi-component surface chemical gradient by means of the ‘e-click’ (2 min) of a fluorescein-labelled alkyne followed by a switch of the polarity of the electrodes and performing a further ‘e-click’ (2 min) of a coumarin-labelled alkyne. Scale bar, 200 μm. ( d ) Fluorescence intensity profiles versus distance from the cathode visualizing the resulting dye gradient for different reaction times (raw data, obtained ex situ ). Full size image Figure 4b shows a fluorescence microscopy image of the resulting surface gradient after 4 min reaction time, showing clearly the highest intensity, and thus coverage, near the cathode. Figure 4c shows a fluorescence microscopy image, after overlaying of images made using the green and blue filters, of a bi-component surface chemical gradient by means of the ‘e-click’ (2 min) of first a fluorescein-labelled alkyne, followed by a switch of the polarity of the electrodes and performing a further ‘e-click’ (2 min) of a coumarin-labelled alkyne. This shows the chemical stability of the azide, even after the reaction, and the versatility of the system. Figure 4d shows fluorescence intensity profiles versus distance to the cathode of a representative batch of ex situ samples (images are shown online in Supplementary Fig. S8 ) at varying reaction times, showing the increase of coverage upon prolonged reaction times. These profiles confirm that, close to the cathode (high [Cu(I)]), the fluorescence intensity increases more rapidly than near the anode (low [Cu(I)]). As a control experiment, a sample was exposed to the same reaction conditions, but without Cu(II) present in the solution. As expected, no reaction occurred ( Supplementary Fig. S9 ). The fluorescence data of the e-click, shown in Fig. 4d versus distance, was plotted versus time, shown in Fig. 5a , as a function of the distance from the cathode. 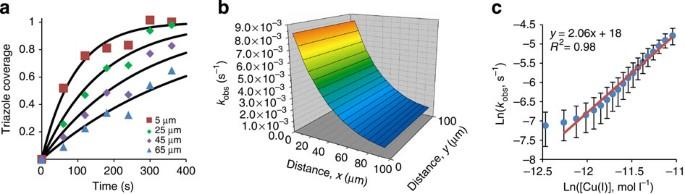Figure 5: Reactivity mapping of the e-click reaction. (a) Data and exponential fits (I(t)=1−e-kobst) of the surface-confined e-click reaction at some characteristic distances from the cathode (high [Cu(I)]) for a single batch of samples. (b) A three-dimensional reactivity map of the e-click reaction kinetics showing thekobsvalues (averaged over several batches of samples) mapped in space in between a cathode (left, ending atx=0) and an anode (right, starting atx=100). (c) Rate order plot of ln(kobs) versus modelled ln([Cu(I)]) values showing a second-order rate dependence on Cu(I). Figure 5a shows representative graphs of the fitted data at four specific distances. These time traces were fitted to the following exponential function: Figure 5: Reactivity mapping of the e-click reaction. ( a ) Data and exponential fits ( I(t) =1− e - k obs t ) of the surface-confined e-click reaction at some characteristic distances from the cathode (high [Cu(I)]) for a single batch of samples. ( b ) A three-dimensional reactivity map of the e-click reaction kinetics showing the k obs values (averaged over several batches of samples) mapped in space in between a cathode (left, ending at x =0) and an anode (right, starting at x =100). ( c ) Rate order plot of ln( k obs ) versus modelled ln([Cu(I)]) values showing a second-order rate dependence on Cu(I). Full size image where I is the normalized fluorescence intensity at time t (s) and k obs is the rate constant (s −1 ). In this way, we explicitly attempt to fit the complete intensity curves, instead of, for example, fitting only the linear initial parts, to provide a comprehensive model description of all data points regardless whether low or high conversion is reached. Because the alkyne in solution is present in excess, a first-order dependence on surface-bound azide is expected as well as a second-order dependence on [Cu(I)] [37] . Because at each specific distance from the cathode we assume [Cu(I)] to be constant, which is supported by the fact that the [Cu(I)] gradient is relatively stable after 60 s as indicated by modelling ( Supplementary Fig. S10 ) and amperometric I - t measurements ( Supplementary Fig. S11 ), the asymptotic enhancement of fluorescence is directly correlated with the decrease in [azide] and concomitant increase in [triazole] at the surface. Therefore, k obs is assumed to be the pseudo first-order (in [azide]) rate constant of the e-click reaction. Figure 5b shows the resulting reactivity map of the e-click data, with the spatial parameters retained, showing the average k obs versus distance from the cathode ( x axis) and along the cathode (y axis). Supplementary Fig. S12 shows the average pseudo first-order rate constants with s.d. Because Cu(I) is generated at the cathode, k obs is, as expected, the highest close to the cathode, with a difference of more than an order of magnitude compared with values near the anode. The parabolic profile observed in Fig. 5b directly visualizes the expected second-order dependence on [Cu(I)]. A finite-element model was set up to estimate the [Cu(I)] gradient and to compare a surface reaction model with the experimental results. The resulting average [Cu(I)] solution gradient, as shown in Supplementary Fig. S13 , was used to determine the rate order of Cu(I) in the e-click reaction. Figure 5c shows a plot of ln( k obs ) versus ln([Cu(I)]), for data of the first 90 μm (see also Supplementary Fig. S14 ; only the last data point was excluded because it was evidently deviating from the linear fit, possibly because of less accurate determination of the conversion in the low-conversion regime). The linear fit of this data results in a slope of 2.06±0.07 ( R 2 =0.98), confirming the second-order dependence on [Cu(I)], which is consistent with the literature [37] . At the moment, our technique has spatial and temporal resolution limits, dictated by the fluorescence microscopy technique used here. The spatial resolution is on the order of 200 nm (at × 100 magnification), whereas the temporal resolution is limited by the minimally needed exposure time (on the order of 100 ms). Also the time needed to obtain a stable solution gradient has a role here, but this can be minimized by bringing the electrodes closer together and reducing the height of the solution on top of the sample effectively turning it into a two-dimensional diffusion case. Of course, with the present system also, other microscopy techniques (for example, total internal reflection microscopy) can potentially be used to increase the lateral resolution and sensitivity. Comparing our technique with scanning electrochemical microscopy (SECM) [38] , it is easier in our case to reach a lateral resolution in the nanometre regime, even in its current state. The temporal resolution, however, is probably worse than that of SECM, especially when going from ultramicroelectrodes to nanoelectrodes, as SECM records electrical current, which can be recorded at extremely high temporal resolution. In an attempt to compare the obtained reaction rates to literature data, the reaction rates cannot be compared with solution studies. For the imine hydrolysis case, one report was found describing a surface reaction [33] , but no reaction rates were determined. However, the timescale of the reaction is roughly the same as ours. In case of the click reaction, a k obs of 0.034 min −1 has been reported [39] . When recalculating k obs from the modelled trend of our data, a k obs value at the same Cu concentration (4 μM) amounts to 0.031 min −1 , which agrees very well and indicates that the reactivities of the click reactions in both systems are very similar. The two chemical reactions probed here, imine hydrolysis and CuAAC, have been analysed to different depths. In the case of the imine hydrolysis, the kinetics is rather complex and the pH dependence may differ for different pH ranges. Experimentally, the pH gradient is not linear, also not when translated in a [H + ] gradient, in particular not near the anode at which the reaction takes place, which may be due to the presence of the buffer. Moreover, the distance range at which the imine hydrolysis takes place is so narrow (only a few micron) that we decided not to attempt a similarly rigorous kinetic treatment as done for the CuAAC case. In conclusion, we show an electrochemical method for the fabrication of micron-scale surface gradients. These gradients are used to study the chemical reactivity of surface reactions in a highly parallel manner. Data is visualized directly as a spatial variation of an electrochemically controlled reaction parameter. It appears possible to derive the Cu(I) reaction order for the CuAAC reaction. As a proof of principle, 1D gradients are used and the detection was done with a fluorescence microscope, but this can potentially be extended to orthogonal gradients, varying two parameters in one experiment, and other surface-characterization techniques (that is, Raman spectroscopy) to remove the constraint of a fluorescent dye present. Furthermore, this method can also be extended to investigate the influence of substrate or reagent concentration by a static surface or solution gradient, respectively. It may even be possible to study reactions in a dynamic fashion, by controlling the solution gradient in time. Optimal use of the method of reactivity mapping will allow the study of a wide range of reactions in which one or more reaction parameters are varied in space and time, while it is envisioned that this method gives the possibility of identification of chemically reactive sites with high spatial resolution. Materials The following materials and chemicals were used as received without further purification: 11-bromoundecyltrichlorosilane (ABCR), sodium azide, hydrazine hydrate (Sigma Aldrich), 6-fluorescein 5(6)-isothiocyanate (Sigma), chloro-1-hexyne, copper sulfate pentahydrate (Aldrich), potassium phthalimide (Fluka), HMDS (BASF), LOR 5A (MicroChem), Olin OiR 907-17 photoresist, Olin OPD 4262 developer (FujiFilm), rhodamine B ethylenediamine, 5-(aminoacetamido)fluorescein (Invitrogen). Alkyne-modified coumarin was prepared as described previously [40] , whereas the synthesis (see Supplementary Fig. S15 for the synthesis scheme) and characterization of alkyne-modified fluorescein is described in the Supplementary Methods . Measurements Fluorescence microscopy images were taken using an Olympus inverted research microscope IX71 equipped with a mercury burner U-RFL-T as light source and a digital Olympus DR70 camera for image acquisition. Ultraviolet excitation (330 nm≤ λ ex ≤370 nm) and blue emission (410 nm≤ λ em ≤510 nm) was filtered using a Olympus DAPI filter cube. Blue excitation (460 nm≤λ ex ≤490 nm) and green emission (λ em >520 nm) was filtered using the Olympus U-MWB2 filter, whereas green excitation (510≤λ ex ≤550 nm) and red emission (λ em >590 nm) were filtered using the Olympus U-MWG2 filter. All fluorescence microscopy images acquired from the imine hydrolysis were taken with 100 μl of aqueous solution on top. The rest of the fluorescence microscopy images were acquired in air. Electrospray ionization time-of-flight mass spectra were recorded using an LCT Mass spectrometer (Waters/Micromass). 1 H and 13 C NMR spectra were recorded on a Varian Unity (300 MHz) spectrometer. 1 H and 13 C chemical shifts values, measured at 300 and 75 MHz, respectively, are reported as δ (in p.p.m.) using the residual solvent signal as internal standard (7.26 p.p.m. for CDCl 3 and 2.50 p.p.m. for dimethylsulphoxide-d 6 ). The electrical current measurements were done with a Karl Süss probe station connected to a Keithley 4200 Semiconductor Characterization System. The electrochemical reactions were performed using an ES015-10 power supply (Delta Elektronica) with voltage range from 0 to 15 V and current range from 0 to 10 A. Imine hydrolysis The procedure for the formation of aldehyde monolayers was adopted from literature [41] . In short, the procedure went as follows. The glass substrates prepatterned with electrode arrays (see Supplementary Methods for the fabrication recipe) were activated by an oxygen plasma treatment (10 min, 50 mA, <200 mTorr, SPI plasmaprep II). After the activation, the substrates were immersed in 0.1 vol% of 11-(triethoxysilyl)undecanal in dry toluene under argon atmosphere for overnight at room temperature. Following monolayer formation, the electrodes were sonicated in toluene (30 s) and rinsed with toluene and ethanol to remove any excess of silanes, and blown dry with N 2 . Then the substrates were placed in an oven (5 min, 120 °C). The substrates were then functionalized by reacting with 0.1 mM of rhodamine B ethylenediamine in water for more than 30 min (the dye was first dissolved in a few drops of ethanol and further diluted with water). After functionalization, the substrates were rinsed with water, ethanol and dried with N 2 , resulting in a full layer of rhodamine dye attached to the substrate via an imine bond. For performing ‘reactivity mapping’ of the hydrolysis of the imine bond on surfaces, the pH was changed from low (anode) to high (cathode) by the following electrochemical reactions, respectively: This pH gradient was generated by application of a potential difference of 1.6 V. The electrochemical system had a voltage source only. By leaving out a reference electrode, we made sure that the current generated at the anode and cathode are of the same magnitude but with opposite sign [42] , which made sure that the two electrochemical reactions occurring are equal when no side reactions are occurring. This should ensure a stable solution gradient in between the interdigitated electrode array. Fluorescence imaging was done ‘ in situ ’. The reactions were performed in silicone containers (Electron Microscopy Sciences) on top of the electrode array with 100 μl of a solution containing 1 mM buffer, pH 7.1 (NaH 2 PO 4 / Na 2 HPO 4 ) and 100 mM electrolyte (Na 2 SO 4 ). CuAAC The procedure for the formation of azide monolayers was adopted from literature [43] . The glass substrates prepatterned with electrode arrays (see Supplementary Methods for the fabrication recipe) were activated by an oxygen plasma treatment (10 min, 50 mA, <200 mTorr). After the activation, the substrates were immersed in 0.1 vol% of 11-bromoundecyltrichlorosilane in dry toluene under argon atmosphere for 1 h at room temperature. Following monolayer formation, the electrodes were rinsed with toluene and ethanol to remove any excess of silanes, and blown dry with N 2 . The bromide/azide nucleophilic substitution was carried out with a saturated NaN 3 solution in dimethylformamide (DMF) for 48 h at 70 °C. The electrodes were thoroughly rinsed with MilliQ water and ethanol, and blown dry with N 2 . For performing ‘reactivity mapping’ of the electrochemically activated CuAAC reaction on surfaces, the Cu(I) concentration was changed from high (cathode) to low (anode) by the following electrochemical reactions, respectively: This gradient in [Cu(I)] was generated by application of a potential difference of 1.0 V. Reactions with different reaction times were performed in silicone containers on top of the electrode array with 100 μl of a solution containing 1 mM alkyne-modified fluorescein and 1 mM Cu(II)SO 4 in dimethylsulphoxide. After the reaction, the electrodes were quickly rinsed with DMF and ethanol to avoid any further progress of the reaction, and blown dry with N 2 . Before fluorescence characterization, all samples were dipped in a 50 mM borax solution at pH 10 for 1 min to assure the activation of the fluorescein dye. Supplementary Fig. S16 shows the reproducibility of the click gradients. In the case of the bi-component surface chemical gradient, the first gradient (fluorescein) is followed by switch of the polarity of the electrodes and performing a further ‘e-click’ (2 min) of a coumarin-labelled alkyne. Modelling The setup was modelled using the commercial Comsol Multiphysics finite-element software (version 4.3). For a complete description, see the Supplementary Methods and Supplementary Table S1 . Furthermore, Supplementary Figs S17 and S18 show the modelled geometry of the pH and click gradient, respectively, and Supplementary Fig. S19 shows the modelling results of the click reaction. How to cite this article: Krabbenborg, S. O. et al. Reactivity mapping with electrochemical gradients for monitoring reactivity at surfaces in space and time. Nat. Commun. 4:1667 doi: 10.1038/ncomms2688 (2013).